Effect of apolipoprotein genotype and educational attainment on cognitive function in autosomal dominant Alzheimer’s disease Autosomal dominant Alzheimer’s disease (ADAD) is genetically determined, but variability in age of symptom onset suggests additional factors may influence cognitive trajectories. Although apolipoprotein E ( APOE ) genotype and educational attainment both influence dementia onset in sporadic AD, evidence for these effects in ADAD is limited. To investigate the effects of APOE and educational attainment on age-related cognitive trajectories in ADAD, we analyzed data from 675 Presenilin-1 E280A mutation carriers and 594 non-carriers. Here we show that age-related cognitive decline is accelerated in ADAD mutation carriers who also have an APOE e4 allele compared to those who do not and delayed in mutation carriers who also have an APOE e2 allele compared to those who do not. Educational attainment is protective and moderates the effect of APOE on cognition. Despite ADAD mutation carriers being genetically determined to develop dementia, age-related cognitive decline may be influenced by other genetic and environmental factors. Presence of the e4 allele of the apolipoprotein E ( APOE ) gene is associated with increased risk for developing sporadic Alzheimer’s disease (AD) and an earlier age of clinical onset than for individuals without an e4 allele [1] , [2] . However, evidence for an effect of APOE e4 genotype on cognitive function in autosomal dominant AD (ADAD) has been limited and inconclusive. ADAD is genetically determined by mutations on the amyloid precursor protein ( APP ), Presenilin-1 ( PSEN1 ), and Presenilin-2 ( PSEN2 ) genes [3] . The largest known kindred with ADAD due to a single mutation ( PSEN1 E280A) resides in Antioquia, Colombia. Carriers of this mutation have a median age of onset of mild cognitive impairment at 44 years and of dementia at 49 years [4] . Despite the group’s well-characterized trajectory, there is individual variability in disease progression, highlighting the need to identify other genetic and environmental factors which may influence age-related cognitive decline. The role of APOE e4 in this kindred has been inconclusive. In a previous study of 109 PSEN1 E280A mutation carriers, those who had an APOE e4 allele had an earlier age of dementia onset than those who did not [5] . A subsequent study of 71 carriers in the same kindred found no effect of APOE e4, but found that the presence of the e2 allele was associated with delayed clinical onset by approximately eight years [6] . Broader investigations including ADAD carriers from multiple families have reported differences between APP and PSEN1 mutations, which may mask APOE effects in combined analyses, but indicate detrimental effects on cognitive performance and decline in PSEN1 carriers [7] , [8] , demonstrating the importance of additional investigation in a large single kindred. In addition, environmental factors (such as lifestyle, health, and socioeconomic conditions) may influence age-related cognitive trajectories and mitigate genetic risk [9] , [10] , [11] . One such factor is education (often defined as years of formal educational attainment), which has been identified as an important modifiable factor for dementia delay and prevention [12] . Higher educational attainment has been associated with slowed cognitive decline in older adults [13] and lower dementia incidence [14] , indicating educational attainment promotes cognitive resilience in the face of pathology [15] . The reported impact of educational attainment in ADAD, however, is inconsistent. Lower educational attainment was a predictor of cognitive decline in ADAD due to various mutations [7] and of earlier clinical onset in PSEN1 E280A carriers [16] . Unexpectedly, however, lower educational attainment (less than three years) has also been associated with later onset of dementia in carriers of the PSEN1 E280A mutation [5] . Of note, ruralness was independently associated with both lower educational attainment and later age of onset in that sample [5] , which may have contributed to the observed relationship. There have been no reported significant interactive effects between APOE genotype and educational attainment in ADAD to date. Additional investigation in this kindred is required to clarify these discrepant findings. The role of genetic and environmental factors impacting age-related cognitive decline in ADAD are critical to further understand disease progression and to support future prevention and treatment goals. In this study, we aimed to evaluate the influence of APOE genotype on cognitive function in 675 PSEN1 E280A carriers and 594 non-carrier family members, and secondarily explore whether educational attainment may be protective and moderate the relationship between APOE and cognitive function. We hypothesized that presence of the e4 allele would be associated with accelerated onset of cognitive impairment, presence of the e2 allele would be associated with delayed cognitive impairment, and that higher educational attainment would be protective against cognitive impairment. Consistent with our hypotheses, in this work we show that the onset of age-related cognitive decline is accelerated in PSEN1 E280A mutation carriers who are also APOE e4+ compared to those who are APOE e4− and delayed in those who are APOE e2+ compared to APOE e2−. Further, we find that educational attainment is protective and moderates the effect of APOE on cognition in PSEN1 carriers. 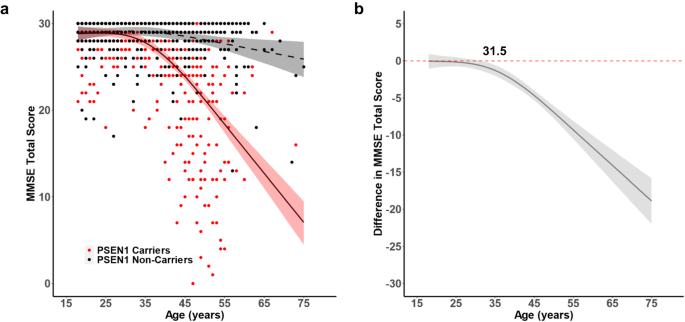Fig. 1: Age-related trajectories of cognitive impairment inPSEN1E280A mutation carriers and non-carriers. aCross-sectional MMSE scores ofPSEN1E280A mutation carriers (red) and non-carriers (black) as a function of age.bDifferences in MMSE score betweenPSEN1E280A mutation carriers and non-carriers as a function of age. MMSE score declines in mutation carriers begins to differ from non-carriers at 31.5 years. The shaded areas of each plot represent the 99% credible intervals around the model estimates drawn from the distributions of model fits derived by the Hamiltonian Markov chain Monte Carlo analyses. MMSE Mini Mental State Examination. Source data are provided as a Source Data file. Sample characteristics Sample characteristics are presented in Table 1 . Of the 675 PSEN1 E280A mutation carriers, 141 were APOE e4+ and 534 were APOE e4−. The APOE e4+ and e4− PSEN1 E280A mutation carriers did not differ in age ( p = 0.64) or sex ( p = 0.89), and they did not differ in MMSE score ( p = 0.52) when collapsing across age. PSEN1 E280A mutation carriers who were also APOE e4+ had on average more years of educational attainment than those who were APOE e4− ( p = 0.02). Of the 594 PSEN1 E280A mutation non-carriers, 148 were APOE e4+ and 446 were APOE e4−. Within these non-carriers, APOE e4+ and e4− individuals did not differ in age ( p = 0.42), sex ( p = 0.23), educational attainment ( p = 0.42), or MMSE score ( p = 0.82). Table 1 Participant demographics stratified by PSEN1 and APOE genotype Full size table Age-related cognitive function by PSEN1 and APOE e4 genotype We first estimated the age-related trajectory of cognitive impairment, measured through MMSE total score, using the Hamiltonian Markov chain Monte Carlo method in PSEN1 E280A mutation carriers and non-carriers, irrespective of APOE genotype. MMSE was negatively associated with age in PSEN1 carriers and significantly differentiated carriers from non-carriers at 31.5 years (Fig. 1 ). Fig. 1: Age-related trajectories of cognitive impairment in PSEN1 E280A mutation carriers and non-carriers. a Cross-sectional MMSE scores of PSEN1 E280A mutation carriers (red) and non-carriers (black) as a function of age. b Differences in MMSE score between PSEN1 E280A mutation carriers and non-carriers as a function of age. MMSE score declines in mutation carriers begins to differ from non-carriers at 31.5 years. The shaded areas of each plot represent the 99% credible intervals around the model estimates drawn from the distributions of model fits derived by the Hamiltonian Markov chain Monte Carlo analyses. MMSE Mini Mental State Examination. Source data are provided as a Source Data file. Full size image We then estimated the age-related trajectory of cognitive impairment as a function of APOE e4 genotype separately in PSEN1 E280A mutation carriers and non-carriers. The cognitive trajectories of APOE e4+ and e4− PSEN1 E280A mutation carriers diverged at 44.3 years, approximately the median age of onset of mild cognitive impairment in this kindred [4] (Fig. 2A, B ). In contrast, the age-related cognitive trajectories of APOE e4+ and e4− PSEN1 E280A mutation non-carriers did not diverge (Fig. 2C, D ). To supplement these analyses, age of clinical onset was compared in a subset of PSEN1 mutation carriers who had converted to MCI or dementia. Consistent with the prior findings, PSEN1 mutation carriers who were also APOE e4+ had earlier ages of clinical onset compared to those who were APOE e4− (Supplementary Table 1 ). Fig. 2: Age-related trajectories of cognitive impairment in PSEN1 E280A mutation carriers and non-carriers stratified by presence or absence of APOE e4. a Cross-sectional MMSE scores of PSEN1 E280A mutation carriers who are APOE e4+ (red) and APOE e4- (black) as a function of age. b Differences in MMSE score between APOE e4+ and e4− PSEN1 E280A mutation carriers as a function of age. MMSE score declines in APOE e4+ PSEN1 E280A mutation carriers begins to differ from APOE e4− PSEN1 E280A mutation carriers at 44.3 years. c Cross-sectional MMSE scores of PSEN1 E280A mutation non-carriers who are APOE e4+ (red) and APOE e4− (black) as a function of age. d Differences in MMSE score between APOE e4+ and e4- PSEN1 E280A mutation non-carriers as a function of age. MMSE score does not differ between APOE e4+ and e4− PSEN1 E280A mutation non-carriers in this age range. The shaded areas of each plot represent the 99% credible intervals around the model estimates drawn from the distributions of model fits derived by the Hamiltonian Markov chain Monte Carlo analyses. MMSE = Mini Mental State Examination. Source data are provided as a Source Data file. Full size image Role of educational attainment on cognition in PSEN1 E280A carriers Years of educational attainment was examined as a protective and potentially modifying factor of the relationship between APOE e4 and cognitive function using separate linear regressions for PSEN1 E280A mutation carriers and non-carriers. Within PSEN1 E280A mutation carriers, being APOE e4+ was associated with lower MMSE scores compared to APOE e4− ( β = −3.37, p = 0.001). Irrespective of APOE genotype, higher educational attainment was associated with higher MMSE scores ( β = 0.41, p < 0.001). There was also a significant interaction between APOE e4 and years of educational attainment ( β = 0.32, p = 0.005; Fig. 3a ) such that the negative effect of APOE e4+ was attenuated as years of educational attainment increased. In other words, higher levels of educational attainment mitigated the additional risk conferred by the presence of at least one e4 allele in PSEN1 E280A carriers. Fig. 3: Cognitive function by years of educational attainment in PSEN1 E280A mutation carriers stratified by APOE genotype. Mini Mental State Examination scores plotted by years of formal educational attainment in PSEN1 E280A mutation carriers stratified by a APOE e4 genotype (red: APOE e4+; black: APOE e4−) and b APOE e2 genotype (red: APOE e2−; black: APOE e2+). Plots show regression line with shaded standard error bands. MMSE = Mini Mental State Examination. Source data are provided as a Source Data file. Full size image In non-carriers of the PSEN1 E280A mutation, there was no significant effect of APOE e4 on MMSE score ( β = −0.17, p = 0.66), but there was a significant main effect of educational attainment ( β = 0.16, p < 0.001) such that higher educational attainment was associated with higher MMSE scores. There was no interaction between APOE e4 and educational attainment ( β = −0.003, p = 0.94). Age-related cognitive function by PSEN1 and APOE e2 genotype Our findings suggest that within PSEN1 E280A carriers, age-related cognitive decline begins earlier in those who are APOE e4+ than for those with other APOE genotypes, including those who are homozygous e3 and e2+. Because presence of the e2 allele has been associated with delayed clinical onset in this kindred [6] , we sought to examine the association between APOE e2 and cognition in our current sample. 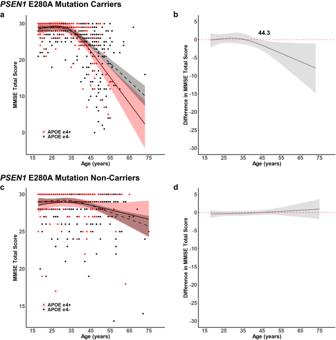Fig. 2: Age-related trajectories of cognitive impairment inPSEN1E280A mutation carriers and non-carriers stratified by presence or absence ofAPOEe4. aCross-sectional MMSE scores ofPSEN1E280A mutation carriers who areAPOEe4+ (red) andAPOEe4- (black) as a function of age.bDifferences in MMSE score betweenAPOEe4+ and e4−PSEN1E280A mutation carriers as a function of age. MMSE score declines inAPOEe4+PSEN1E280A mutation carriers begins to differ fromAPOEe4−PSEN1E280A mutation carriers at 44.3 years.cCross-sectional MMSE scores ofPSEN1E280A mutation non-carriers who areAPOEe4+ (red) andAPOEe4− (black) as a function of age.dDifferences in MMSE score betweenAPOEe4+ and e4-PSEN1E280A mutation non-carriers as a function of age. MMSE score does not differ betweenAPOEe4+ and e4−PSEN1E280A mutation non-carriers in this age range. The shaded areas of each plot represent the 99% credible intervals around the model estimates drawn from the distributions of model fits derived by the Hamiltonian Markov chain Monte Carlo analyses. MMSE = Mini Mental State Examination. Source data are provided as a Source Data file. 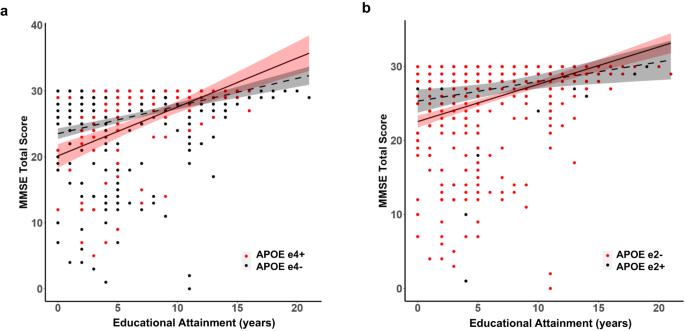Fig. 3: Cognitive function by years of educational attainment inPSEN1E280A mutation carriers stratified byAPOEgenotype. Mini Mental State Examination scores plotted by years of formal educational attainment inPSEN1E280A mutation carriers stratified byaAPOEe4 genotype (red:APOEe4+; black:APOEe4−) andbAPOEe2 genotype (red:APOEe2−; black:APOEe2+). Plots show regression line with shaded standard error bands. MMSE = Mini Mental State Examination. Source data are provided as a Source Data file. Of the 675 PSEN1 E280A mutation carriers, 102 were APOE e2+ and 573 were APOE e2− (Supplementary Table 2 ). The APOE e2+ and e2− PSEN1 E280A mutation carriers did not differ in age ( p = 0.20), sex ( p = 0.65), educational attainment ( p = 0.69), or MMSE score ( p = 0.37). Of the 594 PSEN1 E280A mutation non-carriers, 73 were APOE e2+ and 521 were APOE e2−, and APOE e2+ and e2− individuals did not differ in age ( p = 0.47), sex ( p = 0.12), educational attainment ( p = 0.70), or MMSE score ( p = 0.66). We first estimated the age-related trajectory of cognitive impairment as a function of APOE e2 genotype separately in PSEN1 E280A mutation carriers and non-carriers (Supplementary Fig. 1a, b ). The cognitive trajectories of APOE e2+ and e2− PSEN1 E280A mutation carriers diverged at 41.1 years, such that APOE e2+ PSEN1 carriers had delayed age-related global cognitive decline. Age of clinical onset of the MCI and dementia converters did not significantly differ between APOE e2+ and e2− genotypes, but the trends were in the hypothesized direction such that APOE e2+ mutation carriers had on average later clinical onset (Supplementary Table 1 ). In PSEN1 E280A mutation non-carriers, the age-related cognitive trajectories of APOE e2+ and e2− individuals did not diverge (Supplementary Fig. 1c, d ). We then assessed the relationships between APOE e2 genotype and educational attainment on global cognitive function. Within PSEN1 E280A mutation carriers, there was a main effect of genotype, such that those who were APOE e2− had lower MMSE scores than those who were APOE e2+ ( ß = −2.78, p = 0.007). Across APOE genotype, higher educational attainment was associated with higher MMSE scores ( ß = 0.26, p = 0.018). Additionally, there was a significant interaction between APOE e2 genotype and educational attainment, ß = 0.24, p = 0.046 (Fig. 3b ), such that higher educational attainment attenuated the negative effect of being APOE e2−. APOE e4 has long been associated with increased risk and earlier age of onset for sporadic AD [1] , [2] , [17] , [18] , [19] , [20] . A rare variant on the APOE e3 allele was found to delay onset of MCI by three decades in a PSEN1 E280A carrier [21] , yet the evidence linking the more common e2 and e4 variants has been mixed [5] , [6] , [22] . Our findings in over 1,000 participants from a single kindred show an added effect of APOE genotype in carriers of the PSEN1 E280A mutation for ADAD, such that APOE e4+ PSEN1 mutation carriers had accelerated onset of age-related cognitive decline compared to APOE e4− PSEN1 mutation carriers. The age-related trajectory of clinical impairment diverged between APOE e4+ and e4− PSEN1 mutation carriers around age 44, approximately the median age of onset of mild cognitive impairment in this kindred [4] . Our results are consistent with a prior study reporting a detrimental effect of APOE e4+ genotype in PSEN1 E280A mutation carriers [5] . A subsequent study of 71 PSEN1 E280A mutation carriers found no effect of APOE e4 genotype, but the relationship was in the expected negative direction [6] , suggesting the study may have been underpowered to detect an effect. Conversely, we found that PSEN1 E280A mutation carriers who were APOE e2+ had delayed onset of age-related cognitive decline, replicating a prior finding from this kindred [6] . The APOE e2 allele has also been associated with delayed onset and protection against cognitive decline in older adults [20] , [23] , [24] . More research is needed to determine how these genetic risk factors contribute to earlier cognitive decline in ADAD. Both APOE e4 and PSEN1 mutations influence accumulation of β-amyloid (Aβ) pathology in the brain [25] , [26] , [27] . This genetic combination may result in earlier or higher pathological burden, but future studies will need to consider age-related trajectories of brain pathology in addition to clinical impairment. Since other mutations causing ADAD also alter Aβ production, similar results might be expected in other ADAD mutations. However, the extent to which these results generalize to ADAD caused by other mutations is uncertain. A study of APP and PSEN1 mutation carriers from six families found no overall effect of APOE e4 on cognitive decline, but in a direct comparison of age-related cognitive decline of APOE e4+ APP and PSEN1 carriers, the APOE e4+ PSEN1 carriers had a steeper decline than the APOE e4+ APP carriers [7] . Additional questions remain about the nuances of APOE genotype in ADAD. It is currently unknown whether the risk is greater in homozygous APOE e4 ADAD mutation carriers than in heterozygous APOE e4 ADAD mutation carriers, as is observed in sporadic AD [2] . This question is particularly challenging to answer in ADAD given the small percentage of homozygous APOE e4 carriers coupled with the small population of ADAD mutation carriers. Observational evidence from a sample of 17 carriers of an APP mutation supports this notion, such that homozygous APOE e4 mutation carriers had the earliest age of onset, followed by the heterozygous APOE e4 mutation carriers, and finally the APOE e2 mutation carriers with the latest onset [28] . In a comparison of early- and late-onset AD, APOE e4 genotype was associated with accelerated cognitive decline in both groups [29] . Coupled with the current results, these findings provide converging evidence that APOE may have similar effects in sporadic and autosomal dominant AD. Furthermore, in sporadic AD, APOE e4 has been associated with better cognitive performance and differing neural activity during young adulthood [30] , [31] , [32] , reflecting possible antagonistic pleiotropy of this genetic risk factor [33] , [34] . Structurally, APOE e4+ adults show greater parahippocampal thickness than APOE e4− adults [35] and differences in white matter integrity that may relate to observed cognitive benefits [36] . Our study only considered age-related cognitive trajectories in adult carriers; however, it is possible that APOE e4 may provide some biological or cognitive benefit in younger PSEN1 carriers (i.e., childhood, akin to young adults in sporadic AD). In fact, PSEN1 carriers in this kindred have greater cortical thickness in childhood than non-carriers, followed by atrophy in adulthood [37] . Studying the influence of both APOE and PSEN1 across the lifespan will enhance our knowledge of the effects of these genes, and, hopefully, provide mechanisms for disease prevention and treatment in the future. Despite the additional risk conferred by APOE e4, our results suggest that educational attainment may be a critical mechanism of cognitive reserve in ADAD, as previously shown in sporadic AD [13] , [14] , [15] . Higher educational attainment was related to higher global cognition in PSEN1 carriers and mitigated the cognitive impairment associated with APOE e4. Prior studies in this kindred have found opposing results, including one in which more years of educational attainment was associated with delayed clinical onset [16] , and one in which higher educational attainment (defined categorically as greater than three years) was associated with lower cognition [5] in PSEN1 mutation carriers. The conflicting results may arise from differences in the samples’ average years of educational attainment, the treatment of educational attainment as a continuous versus categorical variable, or from confounding variables influencing these relationships. In the prior study reporting a detrimental effect of educational attainment, low educational attainment was highly correlated with ruralness, which similarly was associated with later clinical onset [5] . Ruralness, then, may reflect protective factors (e.g., physical activity, environment) that explain the reported positive association of low educational attainment. We similarly found that ruralness was associated with fewer years of educational attainment in our sample, but we did not find an association between ruralness and global cognition (see Supplementary Analysis ). The PSEN1 carriers and non-carriers of our sample are members of the same families, providing a high degree of environmental matching, although additional variables explaining quality rather than quantity of years of educational attainment may contribute to our findings and will be important to consider in future work. Many studies examining education effects in sporadic AD include older adult populations with high levels of educational attainment, with averages often greater than high school or college. This is not representative of the broader population, and there are many conflicting findings in the role of educational attainment on cognitive reserve in older adults [13] , [14] , [38] , [39] . In contrast, our sample included a broad range of educational attainment. Our results indicate that low levels of formal educational attainment, in particular, confers greater risk. As such, programs to increase early years of education may be particularly important as preventative measures, supported by the inclusion of education as one of the 12 modifiable risk factors for dementia in the most recent Lancet commission [12] . The factors contributing to higher versus lower educational attainment (e.g., socioeconomic status, occupational attainment) as well as the underlying biological mechanisms of this APOE -educational attainment interaction require further study, particularly since higher levels of educational attainment have been associated with lower Aβ in ADAD [40] . A primary limitation of this study is the reliance of single time-point data. Although our participants spanned a broad range of ages, and age is highly linked to clinical progression in this kindred, we cannot speak to individual trajectories of decline with these data. Analysis of longitudinal cognitive decline will further clarify whether APOE influences age of onset, rate of decline, or both. Additionally, despite having one of the largest sample sizes compared to prior literature in ADAD, our study was underpowered to assess potential gene dose-dependent effects of the APOE e4 or e2 alleles (see Supplementary Fig. 2 for visualization of age-related cognitive trajectories). Finally, educational attainment is not the sole environmental factor influencing cognition and clinical progression. More work is needed to further understand the impact of other lifestyle and modifiable factors along with their interactions with genetic makeup. Together, our results highlight the importance of studying additional genetic and environmental risk factors in ADAD populations, with critical implications for future disease prevention and interventions. Future studies can push these questions forward by investigating the biological basis for the additive risk of APOE e4 and PSEN1 mutations and for the protective role of APOE e2, and for the aspects and length of educational attainment that can support cognitive function or reduce the risk of dementia. Inclusion of blood-based biomarkers in such studies characterizing disease progression is necessary to increase access in these populations at risk and to understand the biological mechanisms underlying these findings [41] , [42] , [43] . The answers to these questions will inform how to best implement educational interventions in various communities and whether continuing late life education may provide additional protection. These answers are critical as Aβ- and APOE -based treatments for AD are being investigated [44] , [45] . In conclusion, our results demonstrate that (1) age-related changes in global cognitive function may be accelerated in ADAD mutation carriers who are also APOE e4+ compared to those who are APOE e4−; (2) age-related changes in global cognitive function may be delayed in ADAD mutation carriers who are also APOE e2+ compared to those who are APOE e2−; and (3) higher educational attainment may have a protective effect against cognitive impairment, even in the presence of strong genetic risk factors. Study procedures were approved by the Institutional Review Board of the University of Antioquia in Colombia (21-10-605) and were performed in accordance with the ethical standards of the Declaration of Helsinki. All participants provided informed consent prior to the initiation of study procedures. Participants were compensated for their participation in accordance with the approved guidelines. Study design and participants This cross-sectional study included participants over the age of 18 recruited from the Alzheimer’s Prevention Initiative (API) registry of ADAD, which includes more than 6000 living members of a kindred with a high prevalence of carriers of the PSEN1 E280A mutation (approximately 1200 individuals) [46] . All members of the registry reside in Colombia and have a parent with the PSEN1 E280A mutation but are blind to their own genetic status. In total, 675 PSEN1 E280A mutation carriers (370 female, 305 male) and 594 mutation non-carriers (332 female, 262 male) were included in these analyses. Neuropsychological assessments were performed at the University of Antioquia in Colombia. Participants completed a clinical interview and the Mini Mental State Examination (MMSE), administered in Spanish, used as a proxy for cognitive impairment. Cognitive data were stored using REDCap (v. 13.1.29). Investigators were blind to participant genetic status during data collection. Genotyping Genomic DNA was extracted from the blood by standard protocols, and PSEN1 E280A characterization was done at the University of Antioquia using methods previously described [47] . Genomic DNA was amplified with the primers PSEN1 -S 5′ AACAGCTCAGGAGAGGAATG 3′ and PSEN1-AS 5′ GATGAGACAAGTNCCNTGAA 3′. We used the restriction enzyme Bsm I for restriction fragment length polymorphism analysis. Each participant was classified as a PSEN1 E280A carrier or non-carrier. APOE genotyping was performed using a Kompetitive Allele Specific PCR–KASP TM assay [48] (LGV Genomics, Beverly, MA). Due to low numbers of homozygous e4 carriers and homozygous e2 carriers (see Table 2 ), each participant was classified based on the presence of at least one e4 allele (e4+) or no e4 alleles (e4−), and separately, based on the presence of at least one e2 allele (e2+) or no e2 alleles (e2−). Twenty-nine participants (13 PSEN1 carriers and 16 non-carriers) were APOE e2/e4 and, therefore, included in both APOE e4+ and APOE e2+ groups. Table 2 Distribution of APOE genotypes for PSEN1 E280A carriers and non-carriers Full size table Statistical analysis All analyses were conducted in R version 4.2.0, modeled separately for PSEN1 E280A carriers and non-carriers. Group differences in continuous variables were assessed using Mann–Whitney U tests due to non-normality, and dichotomous variables were compared using chi-square tests. APOE genotype was included in analyses as a dichotomous variable. Cognitive impairment was measured through MMSE total score (maximum score = 30). Age-related trajectories were derived from cross-sectional MMSE scores modeled using a restricted cubic spline model. Model parameters were estimated using a Hamiltonian Markov chain Monte Carlo method to compare group trajectories (prior = Cauchy distribution, chains = 8, iterations = 10,000, thin = 10). Linear regression was used to estimate the effect of educational attainment on cognition, with MMSE total score as the dependent variable and APOE genotype, educational attainment, and their interaction term as predictors. Educational attainment was included as a continuous variable, representing self-reported total years of formal educational attainment. Self-reported sex was collected for each participant and is presented in demographic tables. Sex was not included in statistical analyses due to no a priori hypotheses about sex differences and sample size limitations of subdividing the participants by PSEN1 genotype, APOE genotype, and sex; however, the proportions of males and females were roughly similar, and there were no differences in sex distributions in the comparison groups of interest, thus we believe results are generalizable to both males and females. Reporting summary Further information on research design is available in the Nature Portfolio Reporting Summary linked to this article.